Enantioselective synthesis of chiral quinohelicenes through sequential organocatalyzed Povarov reaction and oxidative aromatization Heterohelicenes are of increasing importance in the fields of materials science, molecular recognition, and asymmetric catalysis. However, enantioselective construction of these molecules, especially by organocatalytic methods, is challenging, and few methods are available. In this study, we synthesize enantioenriched 1-(3-indol)-quino[n]helicenes through chiral phosphoric acid-catalyzed Povarov reaction followed by oxidative aromatization. The method has a broad substrate scope and offers rapid access to an array of chiral quinohelicenes with enantioselectivities up to 99%. Additionally, the photochemical and electrochemical properties of selected quinohelicenes are explored. Helicenes, which have rigid ortho -fused π-conjugated polycyclic aromatic structures, are important because of their inherent chirality, which arises from their helicity. Because of their distinctive electronic properties, they have been widely investigated for their potential use in the fields of materials science and molecular recognition [1] , [2] , [3] , [4] , [5] , [6] . They can also serve as chiral ligands and catalysts [1] , [7] , [8] , [9] , [10] and have even been used to increase the activity of catalysts for the oxygen evolution reaction [11] . The potential utility of these molecules has triggered extensive investigation of the synthesis of chiral helicenes with novel structures and functional groups. But, conventional acquisition of chiral helicenes rely mainly on the resolution of racemic helicenes by means of chiral resolution reagents or chiral HPLC separation, or asymmetric syntheses enabled by chiral auxiliaries or chiral substrates [12] , [13] , [14] , [15] , [16] , [17] . However, in sharp contrast with central chirality and axial chirality, which are well-studied, helical chirality, and the catalytic enantioselective synthesis of helicenes, remain under-explored (Fig. 1A ). In 1999, Stará et al. realized the first enantioselective synthesis of helicenes, through [2 + 2 + 2] cycloaddition reactions of triple alkynes catalyzed by a chiral nickel complex [18] . Since then, transition-metal-catalyzed enantioselective [2 + 2 + 2] cycloaddition has frequently been used for asymmetric construction of multiple chiral helicenes [19] , [20] , [21] , [22] , [23] , [24] , [25] , [26] , [27] , [28] , [29] . Another effective method for the synthesis of enantioenriched helicenes involves gold-catalyzed enantioselective intramolecular hydroarylation of alkynes [30] , [31] , [32] , [33] , [34] , [35] . Other transition-metal-catalyzed approaches have been reported [36] , [37] , [38] , [39] , including vanadium-catalyzed oxidative coupling of polycyclic phenols [36] and rhodium-catalyzed enantioselective C-H activation/annulation of 1-aryl isoquinoline derivatives and alkynes [38] . Despite these efforts, challenges associated with relatively high catalyst loadings, harsh reaction conditions, and limited substrate scope remain unsolved. Fig. 1: Background introduction and overview of this work. A The development of asymmetric synthesis of central-, axial- and helical- chirality. B Application examples of quino-containing helicenes. C Enantioselective synthesis of quinohelicenes. D Overview of this work. Full size image The great majority of enantioselective syntheses of helicenes involve transition-metal catalysts, and examples using organocatalytic strategies are limited in number (Fig. 1A ). In 2014, List et al. reported enantioselective synthesis of azahelicenes via asymmetric Fischer indole reactions catalyzed by chiral phosphoric acid [40] . Yan et al. accomplished highly enantioselective synthesis of helicenes via vinylidene ortho -quinone methide intermediates with catalysis by chiral bifunctional amides [41] , [42] . In 2020, Bonne and Rodriguez et al. described asymmetric synthesis of dioxa[6]helicenes by a Michael/ O -alkylation heteroannulation process mediated by a bifunctional quinine-derived squaramide organocatalyst [43] . The increasing demand for enantioenriched helicene compounds in various fields has stimulated the development of efficient methods for stereoselective asymmetric synthesis of structurally diverse helicenes, but efficient methods involving organocatalysis would be highly desirable. Of particular interest are quinohelicenes, a subclass of heterohelicenes with potential applications in optoelectronics [9] , [44] , [45] , [46] , [47] , [48] , [49] , [50] , [51] , asymmetric catalysis [7] , [8] , [9] , [52] , and molecular recognition [53] (Fig. 1B ). To date, only two transition-metal-catalyzed syntheses of chiral quinohelicenes have been reported. In 2014, Tanaka et al. [30] reported gold-catalyzed intramolecular hydroarylation of alkynes, but a high catalyst loading (30 mol%) was required, the substrate scope was limited (only two examples were reported), and the enantioselectivity was only moderate (74% ee) (Fig. 1C ). Very recently, Zhu et al. [39] realized the synthesis of chiral quinohelicenes through palladium-catalyzed asymmetric double imidoylative cyclization (Fig. 1C ). It should be noted that the molecules synthesized by these two methods had the quinoline heterocycle in the middle of the polycyclic aromatic structure. There is an urgent need to develop a highly enantioselective method for the synthesis of quinohelicenes with a side quinoline ring. One of the most attractive approaches for the construction of chiral quinoline-containing molecules is the Povarov reaction, which is an excellent method for building ring systems from simple, readily available substrates [54] , [55] , [56] , [57] , [58] , [59] , [60] , [61] , [62] . And, we found that the Povarov reaction catalyzed by lewis acid can be used to construct racemic quinohelicenes, even though which suffered from high catalyst loading and harsh conditions [63] , [64] . Inspired by these works, we speculated that combining a Povarov reaction catalyzed by a chiral Brønsted acid with a subsequent oxidative aromatization would allow the synthesis of chiral quinohelicenes. This approach not only would avoid the use of a transition metal but also would have high step-economy in that the chiral quinohelicene skeleton could be constructed in a one-pot reaction of three easily accessible raw materials. Herein, we report a combination strategy involving a chiral phosphoric acid-catalyzed Povarov reaction and subsequent oxidative aromatization with 1,2-dichloro-4,5-dicyanobenzoquinone (DDQ) to prepare a wide range of chiral quinohelicenes with excellent enantioselectivities (Fig. 1D ). Notably, the obtained quinohelicenes have rich optical properties. The energetic barrier for interconversion between the two enantiomers of helically chiral compounds is known to depend strongly on the number of ortho -fused benzene rings, and helicenes with more than five rings are usually stable. Therefore, to probe the feasibility of our strategy, we calculated the activation energy for racemization of the target quinohelicene, 1-(3-indol)-quino[5]helicene. To our delight, the calculated energy barrier was 36.7 kcal/mol (Fig. 2 ), which is 11.9 kcal/mol higher than the barrier for racemization of the corresponding hydrogen-substituted quino[5]helicene (Supplementary Fig. 4 ). This result indicated that the product we planned to synthesize would be stable at room temperature. With this information in hand, we designed and synthesized benzo[ c ]phenanthren-2-amine 1a from inexpensive, readily available starting materials [36] , [65] , [66] . Fig. 2: Energy barrier to racemization of 1-(3-indol)-quino[5]helicene. The relative Gibbs free energy (kcal/mol) was calculated at the SMD(Toluene)/M06-2X-D3/def2-TZVPP//B3LYP D3(BJ)/def -2-SVP level of theory. Full size image Next, we optimized the conditions for the Povarov reaction of 1a , benzaldehyde ( 2a ), and 3-vinyl-1 H -indole ( 3a ) as model substrates (Fig. 3A ). Initially, the reaction was performed in toluene at 110 °C for 12 h in the presence of 5 mol % ( S )- A1 as the catalyst. Under these conditions, desired tetrahydroquinoline 4a was obtained in 36% yield with 92% ee (entry 1). Subsequently, desired quinohelicene 5a could be obtained in 87% yield with 90% ee by aromatization of 4a . Inspired by this result, we assessed phosphoric acids ( S )- A2 to ( S )- C8 (entries 2–8) and found that ( S )- A5 was optimal, giving 4a with 99% enantioselectivity (entry 5). Fig. 3: Optimization of the reaction conditions. Optimization of conditions for ( A ) the Povarov reaction and ( B ) the oxidative aromatization: a Povarov reaction conditions: 1a (0.05 mmol) and 2a (0.2 mmol) were heated in toluene (1.5 mL) at 110 °C for 12 h; then 3a (0.1 mmol) and CPA* (0.0025 mmol) were added at room temperature (rt), and the reaction was allowed to proceed for 12 h. The dr value for 4a was >20:1. b Isolated yields are reported. c The ee values were determined by high-performance liquid chromatography with a chiral stationary phase. d Oxidative aromatization conditions: 4a (0.05 mmol, 99% ee) and 1,2-dichloro-4,5-dicyanobenzoquinone (DDQ, 0.15 mmol) in solvent (2 mL) were allowed to react at rt for 3 h. e Conversion percentage (cp) = ee 4a /ee 5a × 100%. 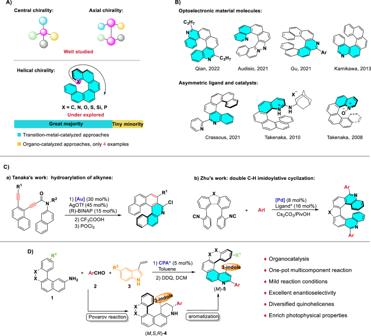Fig. 1: Background introduction and overview of this work. AThe development of asymmetric synthesis of central-, axial- and helical- chirality.BApplication examples of quino-containing helicenes.CEnantioselective synthesis of quinohelicenes.DOverview of this work. Full size image However, the ee for 5a was highly unpredictable when the oxidative aromatization with DDQ was carried out in toluene (Supplementary Table 1 ). To address this issue, we screened various solvents and oxidants for the aromatization step (Fig. 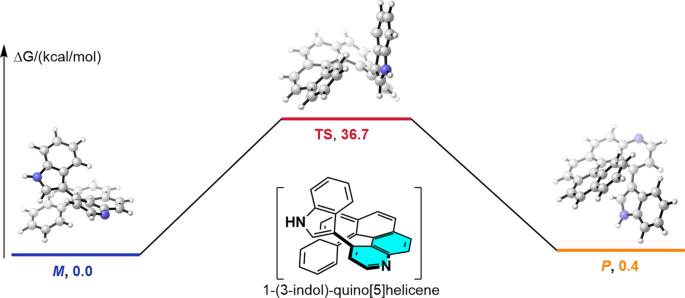Fig. 2: Energy barrier to racemization of 1-(3-indol)-quino[5]helicene. The relative Gibbs free energy (kcal/mol) was calculated at the SMD(Toluene)/M06-2X-D3/def2-TZVPP//B3LYP D3(BJ)/def -2-SVP level of theory. 3B and Supplementary Table 2 ). We were pleased to find that when dichloromethane (DCM) was used as the solvent and oxidize with DDQ, 5a could be obtained in 91% yield with 99% ee with a 100% conversion percentage (Fig. 3B ). To sum up, we obtained the optimal results by carrying out the enantioselective Povarov reaction in toluene to generate 4a and then oxidizing 4a with DDQ in DCM to generate 5a . With optimized conditions in hand, we explored the substrate scope of this reaction. Firstly, various aromatic aldehydes 2 were tested (Fig. 4A ). para -Substituted benzaldehydes 2b – 2j gave corresponding quinohelicene products 5b – 5j in moderate yields (40–67%) with very good enantioselectivities (92–98% ee) regardless of whether the para substituent was electron withdrawing (F, Cl, Br, NO 2 , CF 3 ) or electron donating (Me, OMe, SMe, Ph). We also examined the outcomes of reactions of meta - and ortho -substituted benzaldehydes. These experiments revealed that compounds with electron-donating or electron-withdrawing substituents were well-tolerated, delivering products 5k – 5o with good to excellent enantioselectivities (84–99% ee). Naphthaldehydes were also investigated and found to afford quinohelicenes 5p and 5q with 92% ee and 98% ee, respectively. Furthermore, furfural and 2-thenaldehyde were compatible with the standard reaction conditions and delivered 5r and 5s with 95% ee and 98% ee, respectively. Fig. 4: Scope of the reaction. Scope with respect to ( A ) aromatic aldehyde 2 and ( B ) indole 3 . Reaction conditions: (1) 1a (0.1 mmol) and 2 (0.4 mmol) in toluene (2 mL) were heated at 110 °C for 12 h. After the mixture was cooled to room temperature, 3 (0.2 mmol) and ( S )- A5 (0.005 mmol) were added, and the reaction was allowed to proceed for 12 h. Silica gel column chromatography gave 4 . (2) Reaction of 4 and DDQ (0.3 mmol) in DCM (3 mL) at room temperature for 3 h afforded 5 . Full size image To further explore the substrate scope, we evaluated reactions of 1a and benzaldehyde ( 2a ) with various indoles (Fig. 4B ). We found that indoles with various substituents at C-5 were suitable for this Povarov/oxidation strategy, giving corresponding quinohelicenes 5t – 5w with 98–99% ee. We next investigated reactions of various aromatic amine substrates 1 . Specifically, benzo[ c ]phenanthren-2-amines 1b – 1i were designed and synthesized and allowed to react with 2a and 3a (Fig. 5A ). Gratifyingly, all the tested amines worked well under the optimized conditions, giving the desired products in 45–62% yields with 86–99% ee. Fig. 5: Scope of the reaction. Scope with respect to aromatic amines ( A ), ( B ), ( C ). Reaction conditions: (1) 1 (0.1 mmol) and 2a (0.4 mmol) in toluene (2 mL) were heated at 110 °C for 12 h. After the mixture was cooled to room temperature, 3a (0.2 mmol) and ( S )- A5 (0.005 mmol) were added, and the reaction was allowed to proceed for 12 h. Silica gel column chromatography gave 4 . (2) Reaction of 4 and DDQ (0.3 mmol) and DCM (3 mL) at room temperature for 3 h afforded 5 . Full size image Further exploration of the substrate scope was focused on the helicene skeleton (Fig. 5B ). Chromene-containing quinohelicenes 5aj – 5al were obtained from chromene-containing naphthalen-2-amines 1j – 1l in 46–81% yields with 87–97% ee. Furthermore, dinaphtho[2,1- b :1′,2′-d]furan-2-amine 1 m , which has five rings, was also subjected to the reaction conditions and was found to give quinohelicene product 5am in 46% yield with 94% ee. However, 7H-dibenzo[ c,g ]carbazol-2-amine ( 1n ) failed to provide the corresponding aza-[6]quinohelicene under the standard conditions. The absolute configurations of 5a and 5al were assigned to be M on the basis of X-ray diffraction analysis, and the configurations of the other products were assigned by analogy (Supplementary Fig. 1 and Fig. 2 ). To confirm that our strategy was useful for preparative-scale synthesis, we carried out a 1.0 mmol scale reaction of 1a, 2a , and 3a (Fig. 6A ) and obtained 5a in 57% yield with 95% ee (compare with 99% ee for the small-scale reaction). To illustrate the synthetic utility of the method, we conducted some transformations of 5a (Fig. 6A ). Specifically, alkynyl- and cyano-quino[5]helicenes 6b and 6a , respectively, were obtained in nearly quantitative yields with no loss in optical purity. These chiral products can undergo click reactions and have potential applications in biometrics. To further explore the practicability of the method, we carried out this three-step transformation in one pot (Fig. 6B ). We found that target chiral quinohelicene 5a could be obtained with satisfactory enantioselectivity in toluene, DCM, or ethyl acetate. To our delight, the reaction in ethyl acetate gave 5a in 54% yield with 93% ee. Fig. 6: Synthetic application. Experiments about ( A ) Large-scale reaction and synthetic transformation, and ( B ) One-pot reaction. a The large-scale reaction was conducted under the optimized reaction conditions. b The one-pot reaction was conducted with 1a (0.1 mmol), 2a (0.4 mmol), 3a , and ( S )- A5 (0.005 mmol) in solvent (2 mL) at rt for 24 h; then DDQ (0.5 mmol) was added, and the reaction was allowed to continue for another 3 h. Full size image To investigate the stability of the chiral quinohelicenes, we carried out some racemization experiments (Fig. 7A ). We found that the racemization barriers for 5a and 5aj were 36.3 and 30.2 kcal/mol, respectively, and these values agreed well with the calculated values of 36.4 and 30.6 kcal/mol. The 5.8 kcal/mol difference between 5a and 5aj may have been due to the presence of the sp 3 carbon in 5aj , which made the molecule more flexible. We also found that quino[6]helicene 5am exhibited good configurational stability, and no obvious racemization was observed even after 5 h at 170 °C in 1,2-dichlorobenzene. Additionally, as shown in Fig. 7B , we also explored the stability of the axial chirality of 5a and 5am by DFT calculations. The comparison of the rotation barriers of 5a (11.1 kcal/mol) and 5am (12.3 kcal/mol) suggested the axial chirality of these compounds is extremely unstable at room temperature. Fig. 7: Racemization experiments. Barriers to racemization of ( A ) helical chirality and ( B ) axial chirality. a Experimental relative Gibbs free energy (kcal/mol). b Relative Gibbs free energies were calculated at the SMD(Toluene)/M06-2X-D3/def2-TZVPP//B3LYP D3(BJ)/def −2-SVP level of theory. Full size image To demonstrate the potential applications of the synthesized quinohelicenes, we investigated the photophysical properties of selected molecules (Fig. 8A ). Their fluorescence emission half-lives were determined in DCM, and oxygen-containing compounds 5al and 5am were found to have shorter half-lives than the compounds without oxygen. Notably, the quinohelicenes showed quantum yields ( Φ FL ) up to 26.0%. We also studied the effect of solvent on fluorescence and found that fluorescence gradually increased with increasing solvent polarity and showed a red shift (Fig. 8B ). Moreover, the quantum yield of 5a markedly increased with increasing solvent polarity, from 13.9% in DCM to 43.4% in DMSO (Supplementary Fig. 15 ). Because quinohelicenes exhibit high proton affinities, we studied the optical properties of 5a ·H + in solutions containing 0–50 eq of trifluoroacetic acid. As the amount of acid was increased, the absorption at 240–390 nm gradually weakened; in contrast, that at 400–500 nm increased, and the fluorescence emission peak was markedly red shifted (Fig. 8C ). Fig. 8: Photophysical properties of selected quinohelicenes. A Summary of optical characterization data. B Solvent effect of 5a . C Acid effect of 5a . D Circular dichroic absorption (CD) of M/P - 5a and M/P - 5al . E Circular polarization luminescence (CPL) of M/P - 5a and M/P - 5al . a Measured at a concentration of 1 × 10 −5 M in DCM. b Maximum UV absorption. c Maximum fluorescence wavelength ( λ ex 1 ) and fluorescence lifetime ( λ ex 2 ). 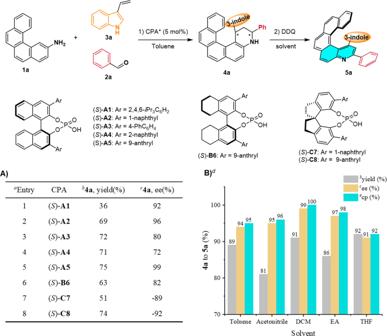Fig. 3: Optimization of the reaction conditions. Optimization of conditions for (A) the Povarov reaction and (B) the oxidative aromatization:aPovarov reaction conditions:1a(0.05 mmol) and2a(0.2 mmol) were heated in toluene (1.5 mL) at 110 °C for 12 h; then3a(0.1 mmol) and CPA* (0.0025 mmol) were added at room temperature (rt), and the reaction was allowed to proceed for 12 h. The dr value for4awas >20:1.bIsolated yields are reported.cThe ee values were determined by high-performance liquid chromatography with a chiral stationary phase.dOxidative aromatization conditions:4a(0.05 mmol, 99% ee) and 1,2-dichloro-4,5-dicyanobenzoquinone (DDQ, 0.15 mmol) in solvent (2 mL) were allowed to react at rt for 3 h.eConversion percentage (cp) = ee4a/ee5a× 100%. d Absolute fluorescence quantum efficiency for absorbance of < 0.1. e Measured for compounds with 99% ee. g abs = Absorption dissymmetry factors; g lum = luminescence dissymmetry factors. Full size image Finally, the chiroptical properties of M - 5a, M - 5ab, M - 5ac, M - 5ae, M - 5ah, M - 5al , and M - 5am , were preliminarily evaluated (Fig. 8A ). The circular dichroism spectra of these quinohelicenes displayed several signals at 230–400 nm and had fine absorption dissymmetry factors ( g abs ); the maximum values for M - 5ab, M - 5ac , and M - 5ae reached −0.0072, 0.0083, and 0.0081 at absorption wavelengths of 390, 393, and 388 nm, respectively. The circular dichroism spectrum of enantiomer P- 5a was the mirror image of the spectrum of M- 5a , and the spectrum of P - 5al was the mirror image of that of M - 5al (Fig. 8D ). Additionally, the simulated CD spectra of the M - 5a enantiomer have a good agreement with experimentally recorded CD spectra of M - 5a . The circular polarized luminescence spectra of M - 5a, M - 5ab, M - 5ac , and M - 5al showed maximum luminescence dissymmetry factors ( g lum ) of 0.0038, 0.0030, 0.0051, and 0.0030 at emission wavelengths of 457, 459, 465, and 465 nm, respectively. Moreover, M - and P - 5a and M - and P - 5al exhibited mirror-image circular polarized luminescence emissions (Fig. 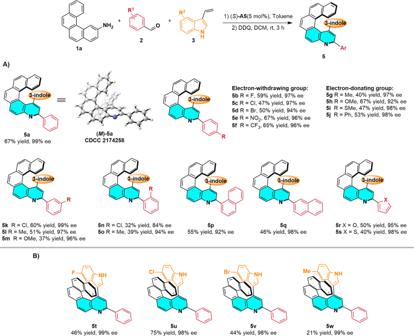Fig. 4: Scope of the reaction. Scope with respect to (A) aromatic aldehyde2and (B) indole3. Reaction conditions: (1)1a(0.1 mmol) and2(0.4 mmol) in toluene (2 mL) were heated at 110 °C for 12 h. After the mixture was cooled to room temperature,3(0.2 mmol) and (S)-A5(0.005 mmol) were added, and the reaction was allowed to proceed for 12 h. Silica gel column chromatography gave4. (2) Reaction of4and DDQ (0.3 mmol) in DCM (3 mL) at room temperature for 3 h afforded5. 8E ). In summary, we have developed a mild, reliable method for multicomponent organocatalytic enantioselective Povarov/aromatization reactions of benzo[ c ]phenanthren-2-amines, aromatic aldehydes, and 3-vinyl-1 H -indoles to prepare highly functionalized quinohelicenes. 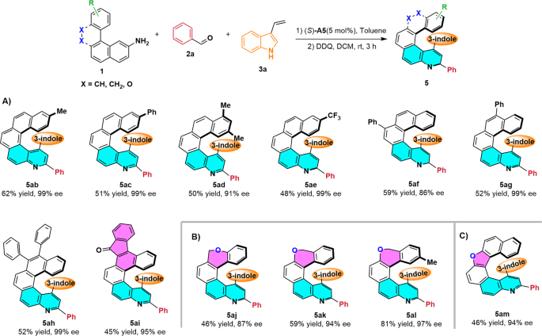Fig. 5: Scope of the reaction. Scope with respect to aromatic amines (A), (B), (C). Reaction conditions: (1)1(0.1 mmol) and2a(0.4 mmol) in toluene (2 mL) were heated at 110 °C for 12 h. After the mixture was cooled to room temperature,3a(0.2 mmol) and (S)-A5(0.005 mmol) were added, and the reaction was allowed to proceed for 12 h. Silica gel column chromatography gave4. (2) Reaction of4and DDQ (0.3 mmol) and DCM (3 mL) at room temperature for 3 h afforded5. 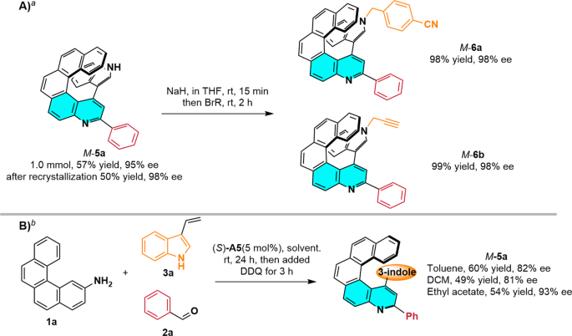Fig. 6: Synthetic application. Experiments about (A) Large-scale reaction and synthetic transformation, and (B) One-pot reaction.aThe large-scale reaction was conducted under the optimized reaction conditions.bThe one-pot reaction was conducted with1a(0.1 mmol),2a(0.4 mmol),3a, and (S)-A5(0.005 mmol) in solvent (2 mL) at rt for 24 h; then DDQ (0.5 mmol) was added, and the reaction was allowed to continue for another 3 h. 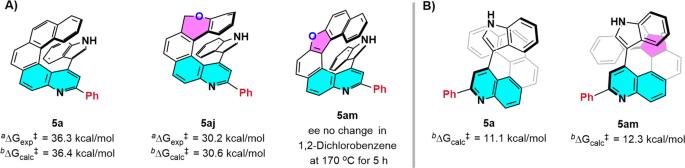Fig. 7: Racemization experiments. Barriers to racemization of (A) helical chirality and (B) axial chirality.aExperimental relative Gibbs free energy (kcal/mol).bRelative Gibbs free energies were calculated at the SMD(Toluene)/M06-2X-D3/def2-TZVPP//B3LYP D3(BJ)/def −2-SVP level of theory. 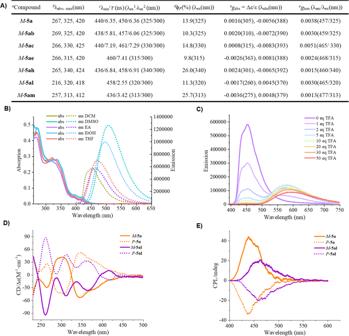Fig. 8: Photophysical properties of selected quinohelicenes. ASummary of optical characterization data.BSolvent effect of5a.CAcid effect of5a.DCircular dichroic absorption (CD) ofM/P-5aandM/P-5al.ECircular polarization luminescence (CPL) ofM/P-5aandM/P-5al.aMeasured at a concentration of 1 × 10−5M in DCM.bMaximum UV absorption.cMaximum fluorescence wavelength (λex1) and fluorescence lifetime (λex2).dAbsolute fluorescence quantum efficiency for absorbance of < 0.1.eMeasured for compounds with 99% ee.gabs= Absorption dissymmetry factors;glum= luminescence dissymmetry factors. The wide substrate scope, good yields, and high enantioselectivities make this a promising method for preparing chiral helicenes, which are widely used for applications in materials science, molecular recognition, and asymmetric catalysis. Moreover, the synthesized quinohelicenes showed enrich photophysical properties, including solvent and acid effects on UV and fluorescence, CD and CPL propeties.